Wide-angle planar microtracking for quasi-static microcell concentrating photovoltaics Concentrating photovoltaics offer a way to lower the cost of solar power. However, the existing paradigm based on precise orientation of large-area concentrator modules towards the Sun limits their deployment to large, open land areas. Here, we explore an alternate approach using high-efficiency microcell photovoltaics embedded between a pair of plastic lenslet arrays to demonstrate quasi-static concentrating photovoltaic panels <1 cm thick that accomplish full-day tracking with >200x flux concentration ratio through small (<1 cm) lateral translation at fixed latitude tilt. Per unit of installed land area, cosine projection loss for fixed microtracking concentrating photovoltaic panels is ultimately offset by improved ground coverage relative to their conventional dual-axis counterparts, enabling a ~1.9x increase in daily energy output that may open up a new opportunity for compact, high-efficiency concentrating photovoltaics to be installed on rooftops and other limited-space urban environments. Optical concentration provides strong cost leverage for high-efficiency photovoltaic (PV) cells [1] . Traditional concentrating PV (CPV) systems rely on large Fresnel lens [2] or mirror-based modules [3] , [4] that must be precisely oriented in the direction of the Sun to maintain high concentration ratio (CR>100). Although simple and effective, this mode of tracking demands robust and often costly mechanical tracking infrastructure to adequately control the movement of large-area CPV modules, especially in windy conditions [5] . Moreover, orientation-based CPV systems have limited siting capability that prevents them from integration in urban environments or on rooftops due to their unwieldy nature and the need for large land area to avoid shading among adjacent systems [6] . Various translation-based CPV tracking strategies have been proposed as an alternative, in which the position of the PV cells and/or multiple concentrator optics are varied laterally with respect to one another. This notion has been explored in the context of mobile freeform optics [7] , [8] and planar waveguide concentrators [9] , [10] ; however, a general difficulty among these approaches is significant deterioration of the concentration ratio at wide (>20° from normal) incidence angles. Since only ~17% of solar illumination incident on a fixed, latitude-tilted panel over the course of a typical 8-h day occurs at incidence <20°, the utility of planar tracking has been limited to date. Here we exploit microscale GaAs PV cells grown in releasable stacks [11] , [12] and integrated with a pair of lenslet arrays in a folded optical path configuration to enable planar microtracking CPV capable of maintaining a >200-fold increase in power output relative to an unconcentrated cell at >70% optical efficiency for incidence angles ranging ±60° at fixed latitude tilt. We demonstrate this approach experimentally for a single microcell using commercial off-the-shelf plano-convex lenses and subsequently extend it to a seven-element small-scale panel prototype featuring three-dimensional (3D)-printed plastic lenslet arrays. This result represents a significant step towards the goal of inexpensive, high efficiency embedded CPV systems that can be integrated on building rooftops and other limited-space urban environments in the form factor of standard fixed panel PV. 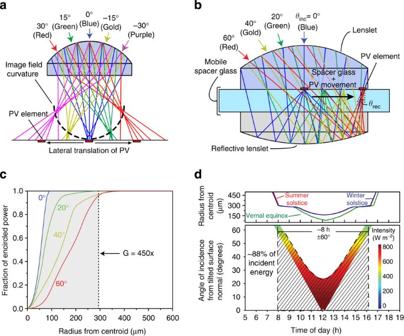Figure 1: Wide-angle microtracking approach. (a) Ray-tracing schematic of a singlet lens used for translation-based solar tracking, where defocusing at wide incidence angle because of Petzval curvature leads to poor performance. (b) Elimination of Petzval curvature through use of a folded optical path, where the focal plane lies in the middle of a dielectric with refractive upper and reflective lower surfaces. In practice, the solar cell (red rectangle) is fixed to a central glass or acrylic sheet that slides between upper and lower lenslets lubricated by index-matching fluid. (c) Fraction of encircled optical power in the focal plane as a function of radius from the intensity maximum for the configuration shown inb. The top and bottom lenses consist of acrylic plastic and have a diameter of 12.7 mm; the simulation is conducted for wavelengthsλ<1.1 μm using the AM1.5D intensity spectrum. (d) Annual range of solar incidence angles (relative to the surface normal) for a latitude-tilted panel over the course of a year in State College, PA, USA. The false colour overlay indicates the approximate direct solar irradiance falling on the panel surface accounting for cosine projection loss. The upper plot displays the calculated focal spot size for the configuration inc, defined as the spot radius encircling 95% of the focal plane optical power, versus time of day for the annual solstices and equinoxes. Wide-angle microtracking Figure 1a illustrates the notion of planar CPV tracking, where a solar cell is translated laterally to follow the focal point of a fixed lens as it moves in response to different solar incidence angles over the course of a day. A major challenge for this approach stems from Petzval curvature of the image plane indicated by the dashed line, where on- and off-axis light concentrates in different axial planes. This effect significantly reduces the optical efficiency of the concentrator for sunlight incident at angles >20° since the focal point no longer coincides with the plane of the solar cell [9] . Figure 1: Wide-angle microtracking approach. ( a ) Ray-tracing schematic of a singlet lens used for translation-based solar tracking, where defocusing at wide incidence angle because of Petzval curvature leads to poor performance. ( b ) Elimination of Petzval curvature through use of a folded optical path, where the focal plane lies in the middle of a dielectric with refractive upper and reflective lower surfaces. In practice, the solar cell (red rectangle) is fixed to a central glass or acrylic sheet that slides between upper and lower lenslets lubricated by index-matching fluid. ( c ) Fraction of encircled optical power in the focal plane as a function of radius from the intensity maximum for the configuration shown in b . The top and bottom lenses consist of acrylic plastic and have a diameter of 12.7 mm; the simulation is conducted for wavelengths λ <1.1 μm using the AM1.5D intensity spectrum. ( d ) Annual range of solar incidence angles (relative to the surface normal) for a latitude-tilted panel over the course of a year in State College, PA, USA. The false colour overlay indicates the approximate direct solar irradiance falling on the panel surface accounting for cosine projection loss. The upper plot displays the calculated focal spot size for the configuration in c , defined as the spot radius encircling 95% of the focal plane optical power, versus time of day for the annual solstices and equinoxes. Full size image Petzval curvature can be minimized by appropriately combining optical elements with positive and negative surface powers as in the case of a common fish-eye lens. In general, however, wide field-of-view lens systems require multiple elements, leading to high reflection loss, excessive size, weight and cost that all run contrary to the goal of an efficient, inexpensive planar concentrator. Alternatively, the Petzval surface can be flattened within a single dielectric by combining refraction from a convex front surface with reflection from a concave rear surface as shown in Fig. 1b to fold the optical path and achieve an intermediate focal plane between the two. To first order, this is understood from the Petzval sum for this configuration, Σ=(1− n )/ nR r +2/ nR m (ref. 13 ), which is nulled when the refractive index, n , together with the refractive ( R r ) and reflective ( R m ) surface radii of curvature satisfy R m / R r =2/( n −1). In contrast to the singlet lens in Fig. 1a , it is immediately evident from ray tracing that the Petzval curvature in the folded path optic of Fig. 1b has been virtually eliminated. The result is a dramatic improvement in the concentrator acceptance angle summarized in Fig. 1c , where a geometric gain of 450, defined as the lens aperture area relative to the spot size enclosing 95% of the power in the focal plane, can be maintained up to ±60° incidence. As shown in Fig. 1d , this acceptance angle range enables the concentrator to operate year-round at this geometric gain for 8 h per day in State College, PA, USA, when fixed at latitude tilt (40.8°) according to solar incidence predicted by the National Renewable Energy Laboratory Solar Position Algorithm [14] . 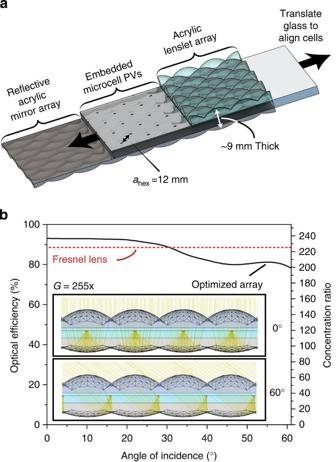Figure 2: Simulated concentrator performance. (a) Schematic illustration of a microtracking microcell CPV panel. An array of microcell photovoltaics is transfer-printed on a central acrylic sheet that tracks by sliding laterally between stationary upper and lower acrylic lenslet arrays lubricated by index matching oil. (b) Simulated absolute optical efficiency of the array ina, defined as the fraction of incident optical power in the AM1.5D solar spectrum (λ<1.1 μm) delivered to the surface of the microcells. The microcell dimensions are 0.7 × 0.7 mm2, whereas the lattice constant of the lenslet array isahex=12 mm, yielding a nominal geometric gainG=255. The maximum lateral translation required at 60° is ±5 mm and the total thickness of the panel is 9 mm. For reference, the simulated optical efficiency of a standard Fresnel lens operating at normal incidence with the same geometric gain is indicated by the red dashed line. The inset shows a cross-sectional ray tracing view of the array at normal (0°) and oblique (60°) incidence angles. Figure 2a illustrates how this configuration can be practically extended in the form of a lenslet array to create a complete CPV panel. Here, matched upper refractive and lower reflective lenslet arrays made of acrylic plastic sandwich, a central (glass or acrylic) sheet with a corresponding transfer-printed array of high-efficiency microcell photovoltaics (loosely defined as side length<1 mm). The central sheet slides freely between the lenslet arrays lubricated by index matching fluid that also functions to eliminate parasitic reflection losses. Hexagonal tiling is chosen because it leads to higher azimuthal symmetry than, for example, a square lenslet array and therefore helps reduce corner-related optical losses. Figure 2: Simulated concentrator performance. ( a ) Schematic illustration of a microtracking microcell CPV panel. An array of microcell photovoltaics is transfer-printed on a central acrylic sheet that tracks by sliding laterally between stationary upper and lower acrylic lenslet arrays lubricated by index matching oil. ( b ) Simulated absolute optical efficiency of the array in a , defined as the fraction of incident optical power in the AM1.5D solar spectrum ( λ <1.1 μm) delivered to the surface of the microcells. The microcell dimensions are 0.7 × 0.7 mm 2 , whereas the lattice constant of the lenslet array is a hex =12 mm, yielding a nominal geometric gain G =255. The maximum lateral translation required at 60° is ±5 mm and the total thickness of the panel is 9 mm. For reference, the simulated optical efficiency of a standard Fresnel lens operating at normal incidence with the same geometric gain is indicated by the red dashed line. The inset shows a cross-sectional ray tracing view of the array at normal (0°) and oblique (60°) incidence angles. Full size image Figure 2b summarizes the simulated performance of this concentrator, optimized for 0.7 × 0.7 mm 2 square microcells at a geometric gain , where a hex and a cell are the hexagonal lattice constant and microcell side length, respectively (that is, G is the ratio of lenslet to microcell area). At normal incidence, the fraction of optical power delivered from the concentrator surface to the microcell array is η opt =0.93, essentially that of a second surface mirror, with losses due only the air/acrylic (no anti-reflection coating is assumed) and acrylic/Ag reflectance. Consistent with Fig. 1b , high-optical efficiency η opt >0.79 is maintained up to θ inc =60° incidence. Defining the flux concentration ratio, CR= Gη opt , as the increase in average intensity received by the microcells relative to that incident on the concentrator surface, therefore results in CR>200 maintained over the entire range of incidence angles, with negligible dependence on azimuth. This result compares favourably with the reference case of a standard acrylic Fresnel lens operating at normal incidence with the same G =255 geometric gain indicated by the red dashed line ( η opt =0.89, CR=225). Optical losses due to shading by the bus line electrical interconnects to each cell are not included in Fig. 2 . Shading loss is estimated in the range 4–11% depending on the bus line width, the thickness of the concentrator stack and the angle of incidence. Off-the-shelf concentrator performance To explore these predictions, a 0.7 × 0.7 mm 2 GaAs microscale photovoltaic cell (thickness ~3 μm) was fabricated and transfer printed onto 1-mm thick B270 glass selected for insertion between two off-the-shelf, 12.7 mm diameter plano-convex BK7 lenses with focal lengths f =15 mm and f =30 mm for the upper and lower elements, respectively. A 150-nm thick layer of Ag was evaporated onto the lower lens surface and the trio was index matched together with oil as shown in Fig. 3a for testing under collimated, broadband illumination from a Xe lamp (see Supplementary Fig. 1 for details). The current–voltage characteristic of a typical microcell under one sun illumination is displayed in Fig. 3b ; performance metrics are detailed in Supplementary Fig. 2 . 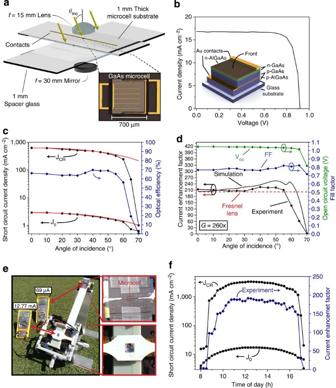Figure 3: Off-the-shelf concentrator testing. (a) Schematic of the testing arrangement for a single 0.7 × 0.7 mm2GaAs microcell using 12.7 mm diameter plano-convex BK7 glass lenses. (b) Current–voltage characteristics measured for a typical microcell under AM1.5D simulated solar illumination. The inset shows a diagram of the device architecture. (c) Short-circuit current density measured under collimated Xe lamp illumination as a function of incidence angle for the microcell located in (JCR) and out (J0) of the concentrator (that is, the bare cell), respectively. The red lines indicate the cosine projection loss relative to normal incidence. Optical efficiency on the right-hand axis represents the fraction of incident power delivered to the microcells and is calculated as described in the text. (d) Simulated and measured current enhancement factors together with the microcell fill factor and open circuit voltage (in the concentrator) as a function of incidence angle. The red dashed line indicates the current enhancement obtained for the same microcell at normal incidence using an acrylic Fresnel lens with the same 12.7 mm diameter aperture size. (e) Photograph showing the concentrator outdoor testing configuration; the insets provide more detailed views of the concentrator and bare cell reference. (f) Short-circuit current density recorded from the bare and concentrated microcells at 15 min intervals throughout the day on 31 May 2014 in State College, PA, USA; the right-hand axis displays the current enhancement factor. Figure 3: Off-the-shelf concentrator testing. ( a ) Schematic of the testing arrangement for a single 0.7 × 0.7 mm 2 GaAs microcell using 12.7 mm diameter plano-convex BK7 glass lenses. ( b ) Current–voltage characteristics measured for a typical microcell under AM1.5D simulated solar illumination. The inset shows a diagram of the device architecture. ( c ) Short-circuit current density measured under collimated Xe lamp illumination as a function of incidence angle for the microcell located in ( J CR ) and out ( J 0 ) of the concentrator (that is, the bare cell), respectively. The red lines indicate the cosine projection loss relative to normal incidence. Optical efficiency on the right-hand axis represents the fraction of incident power delivered to the microcells and is calculated as described in the text. ( d ) Simulated and measured current enhancement factors together with the microcell fill factor and open circuit voltage (in the concentrator) as a function of incidence angle. The red dashed line indicates the current enhancement obtained for the same microcell at normal incidence using an acrylic Fresnel lens with the same 12.7 mm diameter aperture size. ( e ) Photograph showing the concentrator outdoor testing configuration; the insets provide more detailed views of the concentrator and bare cell reference. ( f ) Short-circuit current density recorded from the bare and concentrated microcells at 15 min intervals throughout the day on 31 May 2014 in State College, PA, USA; the right-hand axis displays the current enhancement factor. Full size image Figure 3c presents the short-circuit current density measured for the bare microcell ( J 0 ) together with that integrated in the concentrator stack ( J CR ) as a function of incidence angle. As the photocurrent is directly proportional to absorbed optical power, the difference marks a roughly constant 210-fold increase in the average intensity delivered to the microcell (that is, CR≈210) for incidence angles ranging up to θ inc =55° that is reproduced in simulation as shown in Fig. 3d . As indicated by the red dashed line, this increase is nearly equivalent to that obtained at normal incidence using the bare microcell and a plastic Fresnel lens with the same geometric gain ( G =260). Because the photocurrent angle dependence in each case follows the cosine projection intensity loss designated by the red lines in Fig. 3c , the optical efficiency of the concentrator itself is largely independent of incidence angle. It is estimated on the right-hand axis of Fig. 3c according to η opt ≈ J CR T ac / GJ 0 ‹ T cc ›, where T ac ( θ inc ) is the spectrally averaged Fresnel transmittance from air into the microcell and ‹ T cc › is that from glass into the microcell averaged over the range of angles, θ rec , indicated in Fig. 1b . A potential concern with this method of concentration is non-uniform illumination of the solar cell, which can decrease both open-circuit voltage ( V oc ) and fill-factor (FF) owing to lateral current flow that increases series resistive loss [15] . It is notable then in Fig. 3d that V oc and FF are largely independent of incidence angle for the concentrated microcell, suggesting that the changing illumination profile is not a significant concern. This is presently ascribed to the small microcell dimensions, which reduce the path length and thus voltage drop from lateral current flow. Similarly, microcell dimensions are expected to mitigate thermal loading since the lower absolute power dissipated at each cell location distributes heat over the entire module more effectively; no active cooling was used in any of our measurements. The concentrator stack was subsequently tested outdoors on a sunny day (31 May 2014) tilted at latitude in State College, PA, USA, from 0800 to 1800, h by manually adjusting the translational alignment every 15 min. Figure 3e presents a photograph of the testing arrangement showing the short-circuit current measured for neighbouring microcells located in and out of the concentrator stack. As shown in Fig. 3f , the concentrator operates effectively throughout the day, maintaining a short-circuit current enhancement in the range 150–200x from 0900 to 1700, h. This result is in reasonable qualitative agreement with the enhancement determined under laboratory testing ( Fig. 3d ) and thus, together with V oc and FF that were similarly maintained, equates directly to the increase in power output (see Supplementary Fig. 1 ). 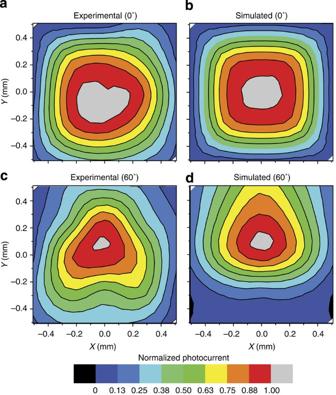Figure 4: Microcell positioning tolerance measurement. Short-circuit current recorded as a function of lateral misalignment between the microcell and the concentrator focal spot for the lens pair experimental configuration inFig. 3. The contour plots ina–ddisplay the photocurrent normalized to its peak (aligned) value at the origin and thus constitute a convolution between the microcell active area and the focal spot intensity distribution. Qualitative agreement is observed between the measurement (a) and ray tracing simulation (b) at normal incidence with a misalignment tolerance of approximately ±0.1 mm. The tolerance narrows to roughly ±0.05 mm for 60° incidence as the focal spot elongates and increases in size for both the measured and simulated data ofcandd, respectively. Contours for the experimental data inaandcare generated from interpolation of an original 5 × 5 grid of data points. Figure 4 explores the illumination profile and microcell positioning tolerance in more detail by mapping the photocurrent as a function of cell position relative to the focal point for normal and oblique incidence angles. These measurements demonstrate an alignment tolerance of approximately ±0.1 mm at θ inc =0° in Fig. 4a that decreases to ±0.05 mm at θ inc =60° in Fig. 4c , consistent with the respective simulations in Fig. 4b,d . The asymmetric nature of the photocurrent map at wide angle results from elongation of the focal spot and is due in part to the use of off-the-shelf spherical lenses; in general, the wide-angle performance can be improved by optimizing towards hyperbolic surface curvature and/or addition of aspheric terms. Figure 4: Microcell positioning tolerance measurement. Short-circuit current recorded as a function of lateral misalignment between the microcell and the concentrator focal spot for the lens pair experimental configuration in Fig. 3 . The contour plots in a – d display the photocurrent normalized to its peak (aligned) value at the origin and thus constitute a convolution between the microcell active area and the focal spot intensity distribution. Qualitative agreement is observed between the measurement ( a ) and ray tracing simulation ( b ) at normal incidence with a misalignment tolerance of approximately ±0.1 mm. The tolerance narrows to roughly ±0.05 mm for 60° incidence as the focal spot elongates and increases in size for both the measured and simulated data of c and d , respectively. Contours for the experimental data in a and c are generated from interpolation of an original 5 × 5 grid of data points. Full size image 3D-printed prototype array Because of the cost and time associated with fabricating custom lenslet arrays via conventional diamond-turning or precision molding techniques, we exploited recent development in 3D-printed optics to fabricate and test a complete, small-scale microcell CPV array. Although 3D printing has begun to revolutionize rapid prototyping in many other fields [16] , [17] , [18] , the goal of printing high-quality optics has remained elusive due to the stringent tolerances imposed on surface error and roughness. The ‘printoptical’ technology [18] employed here aims to address this challenge through controlled buildup and flow of inkjet-printed acrylic plastic, which enables smooth optical surfaces without the need for tooling or post processing. 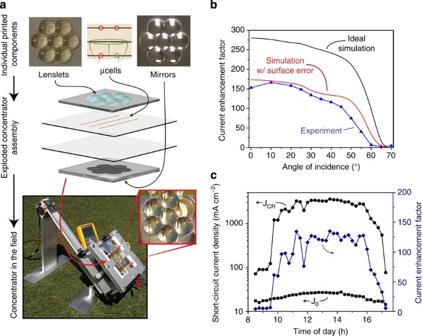Figure 5: Printed lenslet concentrator array. (a) Photographs showing the refractive top and reflective bottom 3D-printed lenslet arrays together with the corresponding layout of GaAs microcells used to construct the concentrator prototype. These components were assembled as illustrated in the diagram to create the full concentrator stack shown in photographs of the outdoor testing configuration at bottom. The cells circled in red (top) were damaged during assembly and excluded (by shorting across them) from measurements; the total photocurrent is the sum of that collected from the bottom right cell and the series-connected middle row of three cells circled in green. (b) Ratio of the short-circuit current recorded from the concentrator stack under collimated Xe lamp illumination relative to that recorded for the bare microcell array outside the concentrator. The measured photocurrent gain is substantially lower than that predicted for this design via ray tracing simulation (solid black line) due to surface error in the printed lenslets. Qualitative agreement is obtained by incorporating Gaussian surface scatter and curvature error into the ray tracing simulation (red line) to model the impact of fabrication defects. (c) Short-circuit current recorded from the prototype array and from the bare reference under full day outdoor testing as shown in (a); the current enhancement ratio is indicated on the right-hand axis. Figure 5a shows the result for a small-scale, seven-element hexagonal lenslet array on acrylic plastic together with a corresponding array of GaAs microcells transfer-printed on a glass substrate. These components were assembled as shown schematically in Fig. 5a to yield a full concentrator stack approximately 1 cm thick with each series-connected row of microcells contacted independently (details of the lenslet optical design and component integration are provided in Supplementary Fig. 3 ). Figure 5b displays the ratio of net short-circuit current measured in and out of the concentrator stack along with that predicted by ray tracing simulation. Here, we observe a peak current enhancement ratio of ~150x that is substantially lower than predicted for the design target. This difference is similar to that measured for a single cell from the array, indicating that surface error in the printed lenslets (as opposed to misalignment of the microcell array positions) is the main factor leading to subpar performance. Although precision interferometry [19] was not available to rigorously characterize the lenslet surfaces, profilometry of a small section of printed lenslet along with the aberration induced in a Gaussian beam and a comparison of simulated concentrator performance (red line) all suggest that relatively large-scale surface error (~20%) is mainly responsible for the lower-than-expected performance (see Supplementary Fig. 4 for details). Figure 5: Printed lenslet concentrator array. ( a ) Photographs showing the refractive top and reflective bottom 3D-printed lenslet arrays together with the corresponding layout of GaAs microcells used to construct the concentrator prototype. These components were assembled as illustrated in the diagram to create the full concentrator stack shown in photographs of the outdoor testing configuration at bottom. The cells circled in red (top) were damaged during assembly and excluded (by shorting across them) from measurements; the total photocurrent is the sum of that collected from the bottom right cell and the series-connected middle row of three cells circled in green. ( b ) Ratio of the short-circuit current recorded from the concentrator stack under collimated Xe lamp illumination relative to that recorded for the bare microcell array outside the concentrator. The measured photocurrent gain is substantially lower than that predicted for this design via ray tracing simulation (solid black line) due to surface error in the printed lenslets. Qualitative agreement is obtained by incorporating Gaussian surface scatter and curvature error into the ray tracing simulation (red line) to model the impact of fabrication defects. ( c ) Short-circuit current recorded from the prototype array and from the bare reference under full day outdoor testing as shown in ( a ); the current enhancement ratio is indicated on the right-hand axis. Full size image Despite the lenslet fabrication error, which could be improved by refining the printoptical process or using molded optics, the initial result in Fig. 5b demonstrates that the requisite microcell patterning and alignment can be achieved, validating the notion of a larger-scale microtracking microcell CPV array. To this point, Fig. 5c presents outdoor testing results for the prototype array conducted in State College, PA, USA, on 1 June 2014, where the concentrator maintains a current enhancement ratio in the range 100–150x relative to the bare reference cell for over 6 h. Cosine projection loss constitutes a fundamental concern for fixed-tilt solar concentration. Whereas polar tracking maintains sunlight at normal incidence, the intensity falling on a fixed panel decreases as the cosine of the incidence angle and thus, per unit panel area, a fixed-tilt system is inherently less efficient than a polar tracking system. This difference is quantified in Fig. 6b , which compares the hourly power output per unit panel area at the vernal equinox in State College, PA, USA, for an optimized microtracking panel with a conventional Fresnel lens at equivalent 255x geometric gain assuming a solar cell efficiency of 30% (refs 20 , 21 , 22 ). Integrated over the day, the polar tracking CPV system delivers approximately 1.5x more energy than the fixed-tilt microtracking system, typical of the difference throughout an entire year. 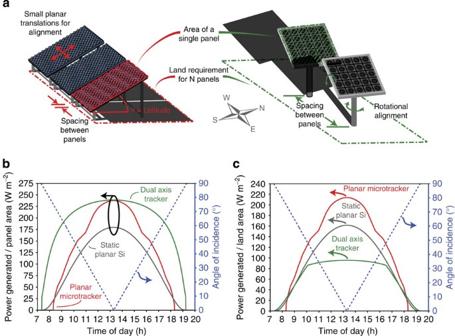Figure 6: Performance comparison. (a) Physical layout of an east–west oriented line of latitude-tilted microtracking panels spaced adjacent to one another. Dual axis tracking conventional Fresnel-based CPV panels shown for comparison must be spaced farther apart to avoid shading one another. (b) Simulated power generation per unit panel area for the microtracking and dual axis systems in (a) along with a latitude-tilted Si photovoltaic module for comparison (gray line). The spacing between dual axis panels is unconstrained and large enough to entirely avoid shading. The dashed line (right-hand axis) designates the solar incidence angle for the fixed-tilt microtracking panels. (c) Power generated per unit installed land area for each system; the dual axis panel spacing in this case is optimized to avoid shading for tilt angles up to 50°. As compared withb, in this case, the planar microtracking system generates nearly twice as much energy on aggregate as the dual axis system over a typical day since more microtracking panels can be located in a given land area without shading. Figure 6: Performance comparison. ( a ) Physical layout of an east–west oriented line of latitude-tilted microtracking panels spaced adjacent to one another. Dual axis tracking conventional Fresnel-based CPV panels shown for comparison must be spaced farther apart to avoid shading one another. ( b ) Simulated power generation per unit panel area for the microtracking and dual axis systems in ( a ) along with a latitude-tilted Si photovoltaic module for comparison (gray line). The spacing between dual axis panels is unconstrained and large enough to entirely avoid shading. The dashed line (right-hand axis) designates the solar incidence angle for the fixed-tilt microtracking panels. ( c ) Power generated per unit installed land area for each system; the dual axis panel spacing in this case is optimized to avoid shading for tilt angles up to 50°. As compared with b , in this case, the planar microtracking system generates nearly twice as much energy on aggregate as the dual axis system over a typical day since more microtracking panels can be located in a given land area without shading. Full size image By the same measure, however, polar tracking panels must be spaced farther apart to avoid shading one another as illustrated in Fig. 6a and thus cosine projection loss is offset when power generation per unit installed land area is the relevant metric. Because microtracking panels can be spaced closely in the east–west direction without shading one another, more power generating capability can be located in a given area of real estate than for polar tracking systems. As shown in Fig. 6c , microtracking PV consequently delivers more power per unit land area over the majority of a typical day, resulting in an approximate 1.9x increase in energy output. Compared with an equivalent installation of Si PV assuming a module efficiency of 18% (grey line), we project a 30% increase in daily energy output delivered by the microcell CPV system. As compared with traditional Fresnel lens CPV systems, embedded microcell microtracking may hold several advantages, particularly for enabling CPV application in urban areas and on rooftops where orientation-based systems have so far been impractical. In addition to improved land use efficiency (cf. Fig. 6 ), microtracking is expected to reduce susceptibility to wind load tracking error and simplify the overall support and tracking infrastructure. At approximately 1 cm thick, microtracking concentration is mechanically simpler and far more compact than previous approaches to fixed panel CPV (See, for example designs by Zettasun Inc. ( http://www.zettasun.com/ ) and Suncycle Holdings, NV ( http://suncycle.nl/ )), with substantially higher optical efficiency owing to the index-matched nature of the concentrator stack. Because lateral displacement of the microcell sheet is limited to ~1 cm (that is, the lenslet pitch) and all movement interfaces are internal and protected, this approach should be mechanically robust, in many respects resembling fixed-panel PV more than traditional CPV. Cost and scalability are also addressed. High-efficiency microcells are now fabricated economically in releasable, multilayer stacks and transfer printing has been demonstrated to pattern and connect them with sub-micrometre precision and high yield over large (Gen 2.5) areas [11] , [21] . Recent cost analysis [23] and commercial success [24] for microcell CPV systems support the potential of this manufacturing approach to be cost-competitive in the photovoltaic marketplace. Simple modes of automated translational microtracking have already been demonstrated [9] and injection molding enables low cost, high-throughput fabrication of plastic lenslet arrays using the same stabilizer additives as existing CPV Fresnel lenses to mitigate ultraviolet-induced yellowing. Long-term colour stability is also documented for index-matching fluids under solar illumination. (See for example refractive index matching liquids such as Code 06350 from Cargille-Sacher Laboratories, Inc. ( http://www.cargille.com/refractivestandards.shtml ).) Mechanical weathering and soiling of the upper lenslet surface are an inevitable concern with plastic optics, although major surface damage could ultimately be resolved by sliding off and replacing the upper lenslet array. Although the detailed impact of thermal expansion and refractive index change arising from climatic variation remains to be investigated, initial estimates suggest a negligible change in focal length and spot size over a 50 °C temperature swing, whereas registration between the microcell and lenslet arrays should be maintained since both are constructed on/from the same plastic. Taken together, our results demonstrate microcell microtracking as a viable route to combine the high efficiency and cost leverage of CPV with the siting versatility and operational robustness of fixed panel PV. Anti-reflection coatings applied to the upper lenslet and microcell surfaces are predicted to maintain full-day optical efficiency between 80 and 95%, whereas global optimization of the lenslet surfaces and microcell size should further increase the concentration ratio. Extension to very high concentration in the range 500–1,000x will likely require a reduction in angular acceptance (for example, ±45°, ~6 h operation per day, see Supplementary Fig. 5 ), which might be economically justifiable given the smaller amount of sunlight sacrificed in the morning and late afternoon cf. Fig. 6c . Supported by the development of multijunction tandem microcells with demonstrated efficiency exceeding 40% [21] , [22] , the embedded microtracking approach described here may provide a new path for efficient, compact and inexpensive photovoltaic power. Simulation Non-sequential ray-tracing simulation was carried out using Zemax optical modelling software accounting for all material absorption/optical constant dispersions and polarization-dependent Fresnel reflections. The geometry of the concentrator stack was simulated and optimized over the AM1.5D solar spectrum in the spectral band 400< λ <1,100 nm accounting for the angular spread of the solar disk to enable implementation with either GaAs or multijunction microcells. In Fig. 6 , the power density of a given panel is calculated as P D ( θ inc )= η cell η opt ( θ inc ) I DNI ( θ inc ), where the net conversion efficiency of the module cell array was conservatively chosen to be η cell =30% (refs 21 , 22 ) and the optical efficiency ( η opt ) is the fraction of light incident on the concentrator that is transmitted to the cells (including the cos( θ inc ) projection loss for the fixed tilt panels). The direct normal irradiance component of the solar spectrum ( I DNI ) was used with an air mass correction to account for intensity changes throughout the day resulting from variation in optical path length through the atmosphere [25] . In Fig. 6c , dual axis tracking panels were spaced for optimal power per unit land area such that shading was avoided for panel tilts up to 50° from the zenith, resulting in a land area increase of [cos(50°)] −1 ~1.55x in the east–west direction relative to microtracking panels spaced adjacent to one another. Latitude-tilted standard Si photovoltaic panels where simulated assuming the AM1.5G solar spectrum, a module efficiency of 18%, incidence angle-dependent Fresnel reflection losses and the same panel-to-panel spacing as the microtracking CPV system. The system comparisons are calculated for a cloudless day at the vernal equinox in State College, PA, USA. Fabrication Microcell PV were grown on GaAs substrates using metal-organic chemical vapour deposition. The cell structure (from bottom to top) includes: the GaAs substrate, a 500 nm Al 0.95 Ga 0.05 As sacrificial layer, a 2,000-nm p-GaAs ( p =3 × 10 19 cm −3 ) bottom contact layer, a 100-nm p-Al 0.3 Ga 0.7 As ( p =5 × 10 18 cm −3 ) back surface field layer, a 2,000-nm p-GaAs ( p =1 × 10 17 cm −3 ) base layer, a 100-nm n-GaAs ( n =2 × 10 18 cm −3 ) emitter layer, a 30-nm n-Al 0.3 Ga 0.7 As ( n =5 × 10 18 cm −3 ) window layer and a 200-nm n-GaAs ( n =1 × 10 19 cm −3 ) top contact layer; electrical contacts consist of 10 nm Cr/200 nm Au. The solar cells are lithographically patterned (size 0.7 × 0.7 mm 2 ), with the Al 0.95 Ga 0.05 As sacrificial layer removed by a hydrofluoric acid (HF)-based solution (ethanol/HF=1.5:1 by volume). Individual solar cells are subsequently transfer printed onto glass substrates using 2-μm-thick SU-8 as an adhesive with electrical interconnects consisting of 10 nm Cr/20 nm Au/1,000 nm Cu/20 nm Au (refs 26 , 27 ). The single-cell concentrator stack ( Fig. 3 ) was constructed using uncoated 12.7 mm diameter BK7 plano-convex lenses (Thorlabs) with focal lengths f =15 mm and f =30 mm for the top and bottom, respectively. The microcells were printed on 1-mm thick glass and sandwiched between the two lenses using index matching fluid (Cargille Labs). The printed lenslet arrays were fabricated by LUXeXcel Inc. on 2- and 3-mm-thick acrylic plastic sheets for the refractive and reflective elements, respectively. These sheet thicknesses are larger than optimal for the optical design but were necessary to avoid substrate bowing due to contraction of the printed acrylic ‘ink’ upon ultraviolet curing. Details are provided in Supplementary Fig. 3 . Characterization The microcell sheet position was controlled manually in all experiments using a pair of crossed translation stages. The entire concentrator/lateral control apparatus was mounted on a sliding track and illuminated from above in order to vary the illumination incidence angle. Measurements were conducted in steady state with a source-measure unit using a laser-driven Xenon lamp (Energetiq) for broadband, collimated illumination (divergence<0.5°) and all-reflective optics to avoid chromatic aberration. Details of the testing arrangement are available in Supplementary Fig. 1 . Owing to the size of the required illumination area (10 cm 2 ) and our limited lamp power, the incident intensity is less than one sun equivalent. Linearity of the microcell photocurrent at high concentration was confirmed separately for illumination intensity exceeding 100 suns ( Supplementary Fig. 2 ). How to cite this article: Price, J. S. et al. Wide-angle planar microtracking for quasi-static microcell concentrating photovoltaics. Nat. Commun. 6:6223 doi: 10.1038/ncomms7223 (2015).